Cathepsin K-mediated notch1 activation contributes to neovascularization in response to hypoxia Cysteine proteases play important roles in pathobiology. Here we reveal that cathepsin K (CatK) has a role in ischaemia-induced neovascularization. Femoral artery ligation-induced ischaemia in mice increases CatK expression and activity, and CatK-deficient mice show impaired functional recovery following hindlimb ischaemia. CatK deficiency reduces the levels of cleaved Notch1 (c-Notch1), Hes1 Hey1, Hey2, vascular endothelial growth factor, Flt-1 and phospho-Akt proteins of the ischaemic muscles. In endothelial cells, silencing of CatK mimicked, whereas CatK overexpression enhanced, the levels of c-Notch1 and the expression of Notch downstream signalling molecules, suggesting CatK contributes to Notch1 processing and activates downstream signalling. Moreover, CatK knockdown leads to defective endothelial cell invasion, proliferation and tube formation, and CatK deficiency is associated with decreased circulating endothelial progenitor cells-like CD31 + /c-Kit + cells in mice following hindlimb ischaemia. Transplantation of bone marrow-derived mononuclear cells from CatK +/+ mice restores the impairment of neovascularization in CatK −/− mice. We conclude that CatK may be a potential therapeutic target for ischaemic disease. Postnatal angiogenesis or neovascularization occurs in response to hypoxia, limb ischaemia or wound healing. Microvascular endothelial cells (ECs) secrete proteinases that permit penetration of the vascular basement membrane as well as the interstitial extracellular matrix during angiogenesis [1] . It is well known that matrix metalloproteinases (MMPs) and serine proteases have essential roles in these processes [2] , [3] . However, recent evidence shows that other proteolytic pathways, such as the cysteine protease cathepsin (Cat) family, are also involved in angiogenesis [4] , [5] . Cats comprise the catalytic classes of serine, aspartate and cysteine peptidases, and exhibit endo- or exopeptidase activities. There is growing evidence for specific intra- and extracellular functions for these lysosomal enzymes, which have been shown to participate in numerous cardiovascular pathogeneses and progressions [6] , [7] , [8] , [9] , [10] . Wang et al . [11] reported that CatS activity controlled the production of matrix-derived angiogenic factors (anti-: canstatin, arresten and tumstatin; pro-: γ2 fragments), revealing a functional role for CatS in angiogenesis and tumour growth. Moreover, recent findings of a few studies show that CatL plays crucial roles in the invasive and functional capacities of endothelial progenitor cells (EPC) in the EPC-mediated neovascularization process [12] , [13] . Cathepsin K (CatK) is essential for extracellular type I collagen and elastin matrix metabolism [14] , [15] . However, no studies thus far have reported on CatK’s roles in tumour- or ischaemia-related angiogenesis. Notch receptors are important regulators of embryonic development and cardiovascular homoeostasis [16] . Among them, endothelial Notch1 has been shown to be critical for vasculogenesis and angiogenesis [17] , [18] . Upon receptor activation, the Notch1 intracellular domain (NICD) is ultimately cleaved by the Presenilin protease (PS1/2) of the γ-secretase complex and translocates to the nucleus associated with RBP-J and mastermind-like proteins to activate the transcription of downstream target genes such as hairy enhancer of split homologue-1 (Hes1), Hes-related repressor (also called Hey) family and angiogenic factors [19] . Thus, γ-secretase strictly controls this terminal cleavage event and Notch1 signal activity. However, the mechanism underlying the proteolytic activation of Notch1 is largely unknown. Here, we report an endothelial CatK-mediated Notch1 activation-based mechanism that plays an essential role in angiogenic actions in response to hypoxia injury. Cysteinyl CatK may be a potential therapeutic target for ischaemic cardiovascular disease. Expression of CatK in ECs Several primary cultured ECs, including human umbilical vein ECs (HUVECs), rat aortic ECs (RAECs) and bovine aortic ECs, had negligible levels of CatK messenger RNA (mRNA) and protein. Exposure to vascular endothelial growth factor (VEGF) causes the accumulation of CatK transcription and translation; the changes were augmented on CoCl 2 -induced hypoxia ( Fig. 1a ). CoCl 2 alone also enhances CatK gene expression. CatK is one of the most potent collagenases [14] , [15] . Acidic gelatin zymography has been used to detect Cat-specific activity [20] . As compared with the control, VEGF with CoCl 2 stimulation exhibited increased collagen degradation; both the CatK-specific inhibitor CatK-II and the nonspecific Cat inhibitor E64 inhibited this activity ( Fig. 1b,c ), suggesting that VEGF with hypoxia enhanced CatK activity. 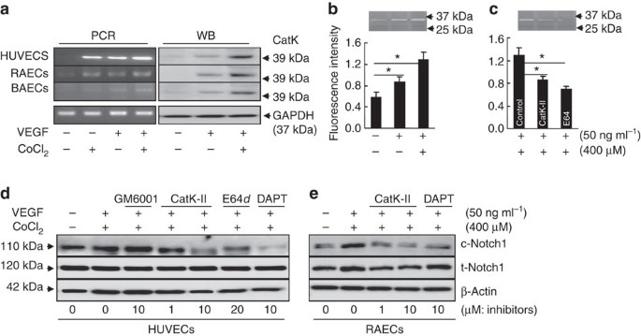Figure 1: Regulation of CatK expression and activity in human umbilical vein endothelial cells (HUVECs), rat aortic endothelial cells (RAECs) and bovine aortic endothelial cells (BAECs). (a–c) Hypoxia enhanced the levels of CatK induced by VEGF in ECs. Cells were induced with 50 ng ml−1VEGF for 24 h at 37 °C in the presence or absence of 400 μM CoCl2. Cell lysates were analysed by PCR, WB and collagenolytic activity assay with or without a specific CatK (CatK-II) or nonspecific (E64d) Cat inhibitor for the levels of CatK gene, protein and activity. Data are means±s.e.m. of three independent experiments performed in triplicate. *P<0.01 by analysis of variance and Tukey’spost hoctests. (d,e) Pharmacological interventions mediated the inhibitory effects on c-Notch1 levels in cultured ECs. Cells were also induced with VEGF under CoCl2-induced hypoxic conditions for 24 h in the presence or absence of various protease inhibitors at the indicated concentrations. The lysates were separately immunoblotted with c-Notch1, t-Notch1 and β-actin antibodies. As we anticipated, ischaemic muscle in vivo had higher levels of VEGF as well as CatK mRNA than nonischemic muscles in CatK +/+ mice ( Supplementary Table 1 ). Figure 1: Regulation of CatK expression and activity in human umbilical vein endothelial cells (HUVECs), rat aortic endothelial cells (RAECs) and bovine aortic endothelial cells (BAECs). ( a – c ) Hypoxia enhanced the levels of CatK induced by VEGF in ECs. Cells were induced with 50 ng ml −1 VEGF for 24 h at 37 °C in the presence or absence of 400 μM CoCl 2 . Cell lysates were analysed by PCR, WB and collagenolytic activity assay with or without a specific CatK (CatK-II) or nonspecific (E64 d ) Cat inhibitor for the levels of CatK gene, protein and activity. Data are means±s.e.m. of three independent experiments performed in triplicate. * P <0.01 by analysis of variance and Tukey’s post hoc tests. ( d , e ) Pharmacological interventions mediated the inhibitory effects on c-Notch1 levels in cultured ECs. Cells were also induced with VEGF under CoCl 2 -induced hypoxic conditions for 24 h in the presence or absence of various protease inhibitors at the indicated concentrations. The lysates were separately immunoblotted with c-Notch1, t-Notch1 and β-actin antibodies. Full size image CatK is involved in c-Notch1 processing in vascular ECs A presenilin/γ-secretase-independent mechanism has been shown to play a partial role in Notch1 signalling transduction. If there are proteases responsible for Notch1 cleavage, we should be able to detect the reduction of cleaved Notch1 (c-Notch1) by treatment with related specific protease inhibitors. To verify this hypothesis, we exposed several types of ECs to VEGF under hypoxia induced by CoCl 2 in the presence or absence of various protease inhibitors at indicated concentrations. γ-Secretase inhibitor (DAPT) was used as a positive control in in vitro experiments. Similar to DAPT, a specific CatK inhibitor (CatK-II) and/or nonspecific Cat inhibitor (E64 d ) had significantly reduced levels of c-Notch1 protein in HUVECs, RAECs and bovine aortic ECs; however, neither MMP inhibitor (GM6001) nor other Cat-specific inhibitors (including CatL inhibitor CatL-V and CatB inhibitor CA-07Me) affected c-Notch1 protein levels ( Fig. 1d,e and Supplementary Figs 1,2 ). Similar to the case with CoCl 2 -induced hypoxia, quantitative western blotting (WB) analysis demonstrated that physical hypoxia also stimulated c-Notch1 processing. The stimulation was augmented when the hypoxia was combined with VEGF; and this effect was still suppressed by CatK-II and E64 d in cultured HUVECs ( Supplementary Fig. 3 ). Thus, among the Cat family, CatK appears to be involved in Notch1 cleavage in ECs under hypoxia. To further address whether the Cat family contributes to Notch1 activation, a series of γ-secretase activity assays with cell lysates and recombinant human Cat (rhCat) was performed in the presence of several specific Cat inhibitors. Expectedly, similar to the case with γ-secretase inhibition, CatK inhibition decreased HUVEC-lysate-associated substrate degradation activity and showed an additive effect by combination with γ-secretase activity inhibition ( Fig. 2a ). As shown in Supplementary Fig. 4 , rhCatK degraded γ-secretase substrate in a time-dependent manner ( Fig. 2b ). γ-Secretase substrate was sensitive to rhCatK in a dose-dependent manner, and this activity was completely inhibited by CatK-II and E64 but was not inhibited at all by a γ-secretase inhibitor L-685,458 (L-685, Fig. 2c,d ) at the concentrations used. Parallel analysis of other Cat family members (rhCatB, rhCatV, rhCaS) and MMP family members (rhMMP-1, rhMT-MMP-1) showed no significant effect ( Fig. 2e , Supplementary Fig. 5 ). Immunofluorescence revealed slight staining signals for the NICD as well as CatK localized in the intramembranous regions of untreated HUEVCs ( Supplementary Fig. 6a ). Interestingly, exposure to VEGF under mechanical hypoxia condition causes the accumulation of c-Notch1 in the nuclei ( Supplementary Fig. 6b ). Therefore, these data further supported our hypothesis that there might be CatK-mediated intramembranous cleavage of Notch1 in vascular cells. In addition, rhCatL showed a certain degradation activity ( Supplementary Fig. 7 ). 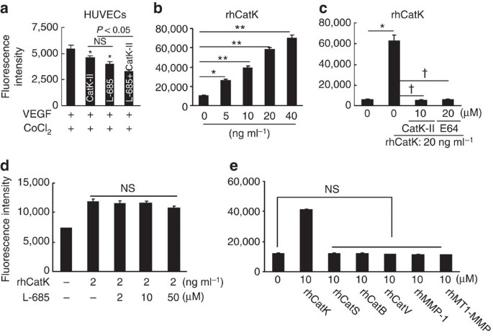Figure 2: CatK-mediated γ-secretase substrate degradation. (a) HUVECs were induced with 50 ng ml−1VEGF for 24 h at 37 °C in the presence of 400 μM CoCl2; the lysate (total protein 200 μg) was incubated with 8 μmol l−1of intramolecularly quenched fluorogenic peptide probe in the presence or absence of CatK-II or L-685, and the CatK activity was then assayed using a plate reader. (b–d) Recombinant human CatK (rhCatK) was incubated with fluorogenic peptide probe for 24 h (pH 6.8) in the presence or absence (b) of a Cat inhibitor (c: CatK-II, E64) and a γ-secretase inhibitor (d: L-685) at the indicated concentrations, followed by fluorescence assay. (e) Various rhCats and rhMMPs were incubated with a fluorogenic probe for 24 h (pH 6.8 for CatK; pH 7.4 for MMP) and then assayed for fluorescence. Data are means±s.e.m. of four to six independent experiments performed in triplicate. *P<0.01,**P<0.001, †P<0.001 by analysis of variance and Tukey’spost hoctests. Figure 2: CatK-mediated γ-secretase substrate degradation. ( a ) HUVECs were induced with 50 ng ml −1 VEGF for 24 h at 37 °C in the presence of 400 μM CoCl 2 ; the lysate (total protein 200 μg) was incubated with 8 μmol l −1 of intramolecularly quenched fluorogenic peptide probe in the presence or absence of CatK-II or L-685, and the CatK activity was then assayed using a plate reader. ( b – d ) Recombinant human CatK (rhCatK) was incubated with fluorogenic peptide probe for 24 h (pH 6.8) in the presence or absence ( b ) of a Cat inhibitor ( c : CatK-II, E64) and a γ-secretase inhibitor ( d : L-685) at the indicated concentrations, followed by fluorescence assay. ( e ) Various rhCats and rhMMPs were incubated with a fluorogenic probe for 24 h (pH 6.8 for CatK; pH 7.4 for MMP) and then assayed for fluorescence. Data are means±s.e.m. of four to six independent experiments performed in triplicate. * P <0.01, ** P <0.001, † P <0.001 by analysis of variance and Tukey’s post hoc tests. Full size image CatK silencing attenuates EC migration and microtubule formation Notch1 signalling regulates EC activity in postnatal angiogenesis [17] . CatK is expressed on proliferating vascular and inflammatory cells during vascular remodelling [5] , and genetic deletion of CatK suppresses cell proliferation and migration infiltration in vivo [21] . Therefore, we assessed whether the blockade of CatK by two small interfering CatK-silencing RNAs (siCatK25 and 26) affects Notch1 activation and EC function. Accordingly, HUVECs were transfected with small interfering RNAs (siRNAs) for 24 h and applied to PCR and western blot analyses. Both siCatKs suppressed not only CatK mRNA and protein but also the levels of c-Notch1, Hes1, Hey1, Hey2, VEGF and p-Akt proteins ( Fig. 3a,b and Supplementary Fig. 8a ). However, two siCatLs had also no effect on Notch1 processing, although it suppressed its expression well ( Supplementary Fig. 8b ). In addition, CatK silencing suppressed HUVEC proliferation ( Fig. 3c ). Simultaneously, nontargeting siRNA and siLam as negative and positive controls, respectively, had no substantial effects on them. Similar to the case with siCatK, pharmacological inhibition of CatK with CatK-II and E64d mimicked these effects ( Supplementary Fig. 3b ). The gain-of-function approach was used to further evaluate CatK’s role in Notch1 processing and its downstream molecule expressions. HUVEC cells were transfected with a CatK plasmid to dramatically increase CatK expression, which resulted in enhanced levels of c-Notch1 protein as well as of Hes1, Hey1 and Hey2 proteins ( Supplementary Fig. 9 ). However, CatS overexpression had no effect on them. As Fig. 3d–f shows, siCatK significantly suppressed VEGF-induced HUVEC migration and tubulogenesis. CatK knockout impaired aortic EC proliferation and sprouting in response to VEGF ( Fig. 3g,h ). Moreover, aorta-ring culture assay showed a reduction in microvessel sprouting in CatK −/− mice ( Fig 4a,c ). 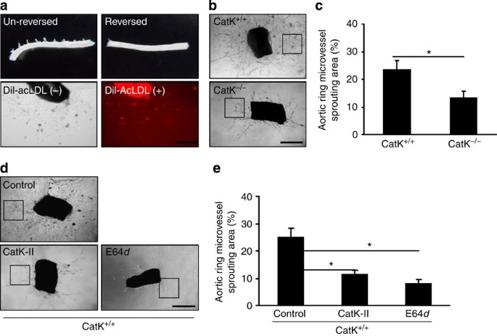Figure 4: Genetic and pharmacological inhibition impairs aorta-derived microvessel outgrowth. (a) Reversed aorta rings (1 mm) were cultured with EBM-2 containing 50 ng mL−1VEGF on type I collagen gel for 7 days, and then microvascular sprouting was characterized by the incorporation of Dil-acLDL (lower panels). (b–e) Aorta rings were induced with 50 ng ml−1VEGF in the presence or absence of Cat inhibitors (CatK-II, E64d) for 5 days. Representative images (b,d) and quantitative data (c,e) for aortic ring microvessel sprouting area (× 200 magnification). The endothelial sprouting area was expressed as a percentage of pixels per image occupied by vessels in the quantitative area. Data are means±s.e.m. of three to five independent experiments performed in triplicate. *P<0.01 by Student’s unpairedt-test or analysis of variance and Tukey’spost hoctests. As anticipated, CatK inhibition by either CatK-II or E64 d dramatically reduced aorta-derived microtubule sprouting in CatK +/+ mice ( Figs 4d,e ). To further verify that outgrowing structures feature capillaries, as previously demonstrated in human aorta-ring assays [22] , we examined sprouting cells by confocal microscopy and immunohistochemistry, and observed the presence of lumens with a mean diameter of 3.6±1.8 μm in a restricted number of outgrowing structures ( Supplementary Fig. 10 ). We previously reported that silencing of Akt, VEGF or Notch1 by each related siRNA blunted the tubulogenic actions of cultured HUVECs and aorta rings [17] , [18] , [23] . 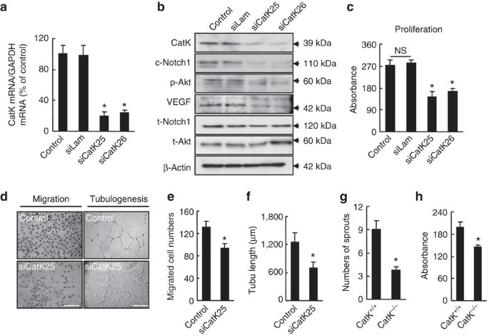Thus, CatK-mediated Notch1 processing appears to represent a mechanism in EC angiogenic actions in response to hypoxic stress. Figure 3: siCatK impairs Notch1 activation and cellular functions in ECs. (a–c) HUVECs were transfected with siRNA targeted to lamin A (as a positive control; siLam) or CatK (using siCatK25 and siCatK26) for 24 h. Cell lysates were analysed by PCR and immunoblotting for the levels of CatK gene (a) and/or other proteins (b: c-Notch1, VEGF, p-Akt); transfected cells were applied to cell proliferation assay (c). Data represent observations from at least three independent experiments. (d–f) Cells transfected with non-siRNA or siCatK25 were applied to migration and tubulogenesis assays. Representative images (d) and quantitative data for migrated cell numbers (e) and tubule length (f). Scale bar, 50 μm. (g,h) CatK deficiency impaired tubulogenic action and proliferation activity. ECs isolated from the aortas of both genotypes of mice were applied to evaluate proliferative activity and tubulogenesis. Data are means±s.e.m. of three to five independent experiments performed in triplicate. *P<0.05 by analysis of variance and Tukey’spost hoctests. Figure 3: siCatK impairs Notch1 activation and cellular functions in ECs. ( a – c ) HUVECs were transfected with siRNA targeted to lamin A (as a positive control; siLam) or CatK (using siCatK25 and siCatK26) for 24 h. Cell lysates were analysed by PCR and immunoblotting for the levels of CatK gene ( a ) and/or other proteins ( b : c-Notch1, VEGF, p-Akt); transfected cells were applied to cell proliferation assay ( c ). Data represent observations from at least three independent experiments. ( d – f ) Cells transfected with non-siRNA or siCatK25 were applied to migration and tubulogenesis assays. Representative images ( d ) and quantitative data for migrated cell numbers ( e ) and tubule length ( f ). Scale bar, 50 μm. ( g , h ) CatK deficiency impaired tubulogenic action and proliferation activity. ECs isolated from the aortas of both genotypes of mice were applied to evaluate proliferative activity and tubulogenesis. Data are means±s.e.m. of three to five independent experiments performed in triplicate. * P <0.05 by analysis of variance and Tukey’s post hoc tests. Full size image Figure 4: Genetic and pharmacological inhibition impairs aorta-derived microvessel outgrowth. ( a ) Reversed aorta rings (1 mm) were cultured with EBM-2 containing 50 ng mL −1 VEGF on type I collagen gel for 7 days, and then microvascular sprouting was characterized by the incorporation of Dil-acLDL (lower panels). ( b – e ) Aorta rings were induced with 50 ng ml −1 VEGF in the presence or absence of Cat inhibitors (CatK-II, E64 d ) for 5 days. Representative images ( b , d ) and quantitative data ( c , e ) for aortic ring microvessel sprouting area (× 200 magnification). The endothelial sprouting area was expressed as a percentage of pixels per image occupied by vessels in the quantitative area. Data are means±s.e.m. of three to five independent experiments performed in triplicate. * P <0.01 by Student’s unpaired t -test or analysis of variance and Tukey’s post hoc tests. Full size image CatK −/− impaired ischaemia-induced vasculogenesis and angiogenesis Because CatK activity was induced by VEGF under hypoxia in ECs, we investigated the functional role of CatK in postnatal neovascularization using a hindlimb ischaemia model. Genetic ablation of CatK expression markedly impaired blood recovery during the follow-up period and capillary formation at day 28 after surgery, indicating that CatK is crucial for ischaemia-induced neovascularization ( Fig. 5 ). To study the molecular mechanism by which CatK controls neovascularization in response to ischaemia, we used immunoblotting to evaluate Notch1 processing and downstream molecule expression and/or phosphorylation in the ischaemic muscles in mice of both genotypes at day 7 after surgery. As shown in Fig. 6a–e and Supplementary Fig. 11 , the levels of c-Notch1, Hes1, Hey1, Hey2, p-Akt, VEGF and Flt-1 were lower in CatK −/− mice than in CatK +/+ mice. Similar to the case with genetic ablation, pharmacological inhibition of CatK by CatK-II also significantly inhibited effects on blood recovery and capillary formation in young mice at day 14 after ischaemia compared with untreated control ( Supplementary Fig 12 ). Figure 6f–g presents a CatK deficiency-related decrease in the γ-secretase substrate probe degradation activity of the fractions extracted from the ischaemic muscles without a change in γ-secretase activity. 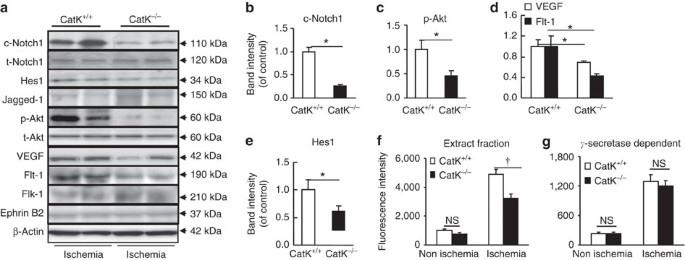Figure 6: The levels of targeted protein in the ischaemic muscles of two experimental groups. (a–e) At day 7 after surgery, equal amounts of total protein extraction were immunoblotted using c-Notch1, t-Notch1, Hes1, Jagged-1, p-Akt, t-Akt, VEGF, Flt-1, Flk-1, Ephrin B2 and β-actin antibodies. Representative immunoblots (a) and quantitative data (b–e) show reduced levels of c-Notch1, Hes1, p-Akt, VEGF and Flt-1 proteins in CatK−/−mice. Data are means±s.e.m. of four independent experiments. (f) Total protein (100 μg) extracted from the ischaemic and nonischemic muscles was incubated with a fluorogenic peptide probe for 24 h (pH 6.8) and then analysed for fluorescence intensity. (g) Enzyme activity assay was performed in the presence of γ-secretase inhibitor (L-685); and γ-secretase-dependent activity was expressed as L-685-induced reduction value. Data are means±s.e.m. of six independent experiments performed in triplicate. *P<0.01,†P<0.05, NS, not significant by Student’s unpairedt-test or analysis of variance and Tukey’spost hoctests. 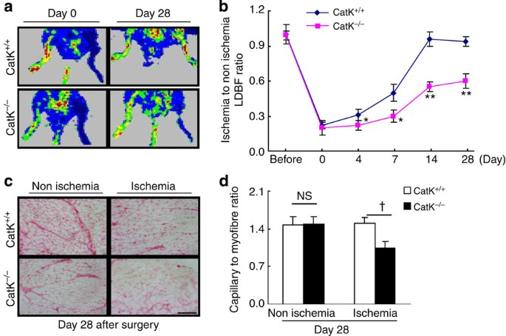We therefore concluded that CatK activity mediates a close link between impaired ischaemia-induced neovascularization and the decline in c-Notch1 processing and downstream signalling transduction in vivo . Figure 5: CatK−/−impaired blood flow recovery and capillary formation in ischaemic muscles of mice. (a) Representative laser Doppler perfusion images showed a low perfusion signal (dark blue) observed in the ischemic hindlimbs of CatK−/−mice and a high signal (red) detected in CatK+/+mice. (b) The ratio of ischaemic to nonischemic laser Doppler blood flow was lower in CatK−/−mice than in CatK+/+mice during the follow-up periods. Data are means±s.e.m. (n=10). *P<0.01, **P<0.01 by two-way repeated measures analysis of variance and Bonferronipost hoctests. (c) Immunohistostaining was performed using GSL-I to visualize capillaries in ischaemic and nonischemic thigh adductor muscle. (d) Quantitative data showed the reduction of capillary density as expressed by the capillary-to-myofibre ratio in ischaemic muscle of CatK−/−mice. Data are means±s.e.m. (n=6).†P<0.01, NS, not significant by analysis of variance and Tukey’spost hoctests. Scale bar, 50 μm. Figure 5: CatK −/− impaired blood flow recovery and capillary formation in ischaemic muscles of mice. ( a ) Representative laser Doppler perfusion images showed a low perfusion signal (dark blue) observed in the ischemic hindlimbs of CatK −/− mice and a high signal (red) detected in CatK +/+ mice. ( b ) The ratio of ischaemic to nonischemic laser Doppler blood flow was lower in CatK −/− mice than in CatK +/+ mice during the follow-up periods. Data are means±s.e.m. ( n =10). * P <0.01, ** P <0.01 by two-way repeated measures analysis of variance and Bonferroni post hoc tests. ( c ) Immunohistostaining was performed using GSL-I to visualize capillaries in ischaemic and nonischemic thigh adductor muscle. ( d ) Quantitative data showed the reduction of capillary density as expressed by the capillary-to-myofibre ratio in ischaemic muscle of CatK −/− mice. Data are means±s.e.m. ( n =6). † P <0.01, NS, not significant by analysis of variance and Tukey’s post hoc tests. Scale bar, 50 μm. Full size image Figure 6: The levels of targeted protein in the ischaemic muscles of two experimental groups. ( a – e ) At day 7 after surgery, equal amounts of total protein extraction were immunoblotted using c-Notch1, t-Notch1, Hes1, Jagged-1, p-Akt, t-Akt, VEGF, Flt-1, Flk-1, Ephrin B2 and β-actin antibodies. Representative immunoblots ( a ) and quantitative data ( b – e ) show reduced levels of c-Notch1, Hes1, p-Akt, VEGF and Flt-1 proteins in CatK −/− mice. Data are means±s.e.m. of four independent experiments. ( f ) Total protein (100 μg) extracted from the ischaemic and nonischemic muscles was incubated with a fluorogenic peptide probe for 24 h (pH 6.8) and then analysed for fluorescence intensity. ( g ) Enzyme activity assay was performed in the presence of γ-secretase inhibitor (L-685); and γ-secretase-dependent activity was expressed as L-685-induced reduction value. Data are means±s.e.m. of six independent experiments performed in triplicate. * P <0.01, † P <0.05, NS, not significant by Student’s unpaired t -test or analysis of variance and Tukey’s post hoc tests. Full size image Vasculogenesis, an important feature of ischaemia-induced neovascularization [24] , depends on various critical steps, including EPC mobilization from the bone niche, transmigration through the vascular basement and proliferation [12] . Because Cats exert widespread substrate specificity, and may thereby influence different processes, we determined the potential involvement of CatK at each individual step. First, we assessed the mobilization of EPCs from the bone marrow (BM) of CatK +/+ and CatK −/− mice. Flow cytometry demonstrated a marked reduction in the number of CD31 + c-Kit + cells in the peripheral blood (PB) of CatK −/− mice at day 10 after ischaemia ( Fig. 7a,b ). However, there was no statistical difference between genotypes in the number of EPC-like CD31 + c-Kit + cells in the BM of mice ( Fig. 7a–b ). Simultaneously, Catk deficiency reduced the levels of c-Notch1, Hes1, Hey1, Hey2 and p-Akt proteins in the c-Kit + cells ( Fig. 7c and Supplementary Fig. 13 ). Moreover, genetic ablation of CatK resulted in a significant change in c-Kit + cell tubule formation, incorporation into the HUVEC network and invasion of the type VI collagen basement membrane ( Fig. 7d–h ). c-Kit + cell proliferation ability was modulated by the pharmacological inhibition of CatK with CatK-II and E64 d ( Fig. 7i ) but not by GM6001-induced inhibition of MMP. Notch1 mediates EC and EPC function in neovascularization [17] . Thus, our data indicate that CatK facilitates EPC mobilization and angiogenic activity to support vasculogenesis associated with Notch1 activation. 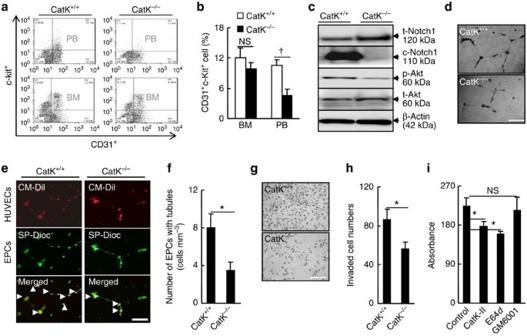Figure 7: CD31+c-Kit+EPC-like cell mobilization is reduced in CatK-deficient mice. (a,b) At day 10 after ischaemic surgery, CD31+c-Kit+was measured by flow cytometry analysis in BM and PB of CatK+/+and CatK−/−mice. Representative images and quantitative data for CD31+c-Kit+EPC-like cell plots and their percentages in BM and/or PB of both genotypes of mice (total 5 × 104cells). Data are means±s.e.m. (n=7).†P<0.05 by analysis of variance (ANOVA) and Tukey’spost hoctests. (c–e) c-Kit+cells isolated by magnetic beads were applied to immunoblotting and tubulogenesis assays; the cells labelled with SP-Dioc were co-cultured with HUVECs labelled with CM-Dil on matrix gel for 24 h. Representative images for immunoblots (c-Notch1, p-Akt) (c), tubule formation (d) and EPC incorporation into the HUVECs network (e). (f) Incorporation of EPC into the HUVECs network was expressed as the number of EPCs with tubules in the quantitative area. (g,h) c-Kit+cells were also applied to invasion and proliferation assays. Representative images and quantitative data for invaded cell numbers. (i) Cell proliferation ability was expressed as absorbance. Data are means±s.e.m. of four independent experiments performed in triplicate. *P<0.01 by Student’s unpairedt-test or ANOVA and Tukey’spost hoctests. Figure 7: CD31 + c-Kit + EPC-like cell mobilization is reduced in CatK-deficient mice. ( a , b ) At day 10 after ischaemic surgery, CD31 + c-Kit + was measured by flow cytometry analysis in BM and PB of CatK +/+ and CatK −/− mice. Representative images and quantitative data for CD31 + c-Kit + EPC-like cell plots and their percentages in BM and/or PB of both genotypes of mice (total 5 × 10 4 cells). Data are means±s.e.m. ( n =7). † P <0.05 by analysis of variance (ANOVA) and Tukey’s post hoc tests. ( c – e ) c-Kit + cells isolated by magnetic beads were applied to immunoblotting and tubulogenesis assays; the cells labelled with SP-Dioc were co-cultured with HUVECs labelled with CM-Dil on matrix gel for 24 h. Representative images for immunoblots (c-Notch1, p-Akt) ( c ), tubule formation ( d ) and EPC incorporation into the HUVECs network ( e ). ( f ) Incorporation of EPC into the HUVECs network was expressed as the number of EPCs with tubules in the quantitative area. ( g , h ) c-Kit + cells were also applied to invasion and proliferation assays. Representative images and quantitative data for invaded cell numbers. ( i ) Cell proliferation ability was expressed as absorbance. Data are means±s.e.m. of four independent experiments performed in triplicate. * P <0.01 by Student’s unpaired t -test or ANOVA and Tukey’s post hoc tests. Full size image MMPs (MMP-2, MMP-9) and cathepsins (CatS, CatL) were recently shown to contribute to pathophysiological angiogenesis [2] , [4] , [12] . We investigated the possibility that CatK deficiency may affect the expression of other proteases, such as Cat and MMP families that might contribute to ischaemia-induced neovascularization. Real-time PCR revealed that, despite the decreases in CatS and MMP-9 gene expression, the genotypes did not differ in their expression of other Cats (CatL, CatB, CatD) and MMPs (MMP-2, tissue inhibitors of MMP −1, −2) in the ischaemic muscles at day 7 after surgery ( Supplementary Table 1 ). Moreover, CatK deletion also exhibited no effects on the expression of Jagged-1 gene. As compared with controls, CatK −/− deficiency lowered the levels of plasma VEGF and interleukin-6 as well as the tissue levels of monocyte chemotactic protein-1 and intracellular adhesion molecule-1 genes. Because activated macrophages have been shown to predominantly produce elastases (including CatS and MMP-9) and VEGF to facilitate ischaemia-induced angiogenesis [2] , [25] , [26] , these decreased inflammation-related actions might also contribute to the impairment of ischaemia-induced neovascularization in these findings. In addition, except for Jagged-1, ischaemic injury increased all targeted molecules in CatK +/+ and CatK −/− mice. Multiple studies have demonstrated that Cats (CatS and CatL) participate in the release of the extracellular matrix and basement membrane-derived growth factors, either by converting them from their latent forms or degrading their associated inhibitors [11] , [27] . Endostatin is a proteolytic fragment of type XVIII collagen generated by several proteases in vivo , including Cats and MMPs. It is possible that CatK or other Cats affect the circulating and local tissue levels of this anti-angiogenic peptide in animals. However, there was no significant difference in the endostatin levels of the ischaemic muscles between mice of the two genotypes (plasma: 17.0±4.5 versus 14.6±5.0; muscle: 57.3±20.9 versus 49.4±17.1 ng ml −1 , P> 0.05 for each group; n =6 for each group; Student's unpaired t -test). On the other hand, it is well known that, among three glycoprotein subunits of laminin-5 (α3, β3 and γ2), γ2 chain-derived fragments promote cancer cell migration, invasion and associated vasculogenesis [28] , [29] . CatS deficiency has been shown to reduce processing of laminin-5 γ2-derived fragments in a mouse tumour model [11] . In contrast, a deficiency of its endogenous inhibitor, cystatin C, promotes tumour growth by enhancing γ2-derived fragment production [26] . WB assays showed no difference in γ2-derived fragment production of ischaemic tissues between CatK +/+ and CatK −/− mice (band intensity: 1.0±0.1 versus. 1.1±0.1, P> 0.05). These observations indicate that CatK has minor effects in endostatin and laminin-5 γ2-fragment production in vivo . Further investigation may be required to assess the contributions of other Cats and MMPs in collagen XVIII- and laminin-5-degradation-related anti-angiogenic endostatin and proangiogenic γ2-fragment production. CatK +/+ BM rescues neovascularization in CatK −/− mice Next, we used BM transplantation assay to further substantiate the specific role of BM-derived CatK in EPCs during vasculogenesis. As shown in Fig. 8a,b , blood flow recovery following hindlimb ischaemia was significantly less impaired in CatK −/− mice receiving CatK +/+ BM-derived c-Kit + cells than in CatK −/− mice receiving CatK −/− BM-derived c-Kit + cells. Consistently, the capillary density and number of CD31 + c-Kit + cells in the PB were significantly higher in mice that had received CatK +/+ BM cells than in mice that had received CatK −/− BM cells ( Fig. 8c–e ). BM transplantation with green fluorescent protein (GFP) mice presented GFP + c-Kit + cells that homed into the ischaemic vasculature at day 14 after surgery ( Fig. 8f ). These data suggested that the lack of CatK especially impairs the functional incorporation of BM-derived EPCs. This may account for the impaired neovascularization capacity of CatK −/− . 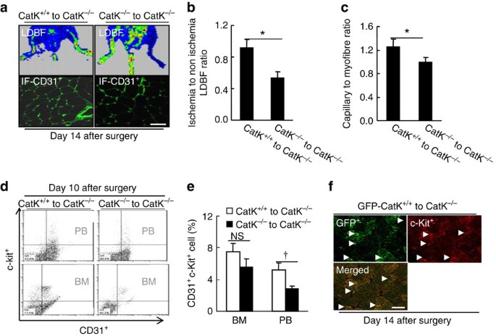Figure 8: Blood flow and capillary formation were improved in CatK−/−mice that received CatK+/+BM-derived EPC-like c-Kit+cells. (a–c) In both genotypes of mice, BM-derived c-Kit+EPC-like c-Kit+cells isolated with microbeads (2 × 106per mouse) were injected directly into the BM cavities of both tibias of irradiated CatK−/−mice (9 Gy) (seeSupplementary Fig. 15) for 40 days. The mice were subjected to ischaemic surgery, after which their blood flow was measured by an laser Doppler blood flow (LDBF) analyser and capillary density was measured by immunofluorescence with fluorescein isothiocyanate-labelled CD31+antibody. Representative images (a) and quantitative data for blood flow recovery (expressed as ischaemia-to-nonischemia LDBF ratio (b); and capillary density (expressed as capillary-to-myofibre ratio (c). Data are means±s.e.m. (n=8). *P<0.05 by Student’s unpairedt-test. (d,e) CD31+c-Kit+measured by FACS analysis in BM and PB of CatK−/−mice that received BM transplantation of both genotypes of mice. Representative images (d) and quantitative data (e) for CD31+c-Kit+EPC-like cell plots and their percentage in BM and/or PB of both genotypes of mice (counted total 5 × 104cells). Data are means±s.e.m. (n=6).†P<0.05 by analysis of variance and Tukey’spost hoctests. (f) At day 14 after ischaemic surgery, fluorescence staining with an anti-c-Kit monoclonal antibody (red) showed EPC homing in to the vasculature of the ischaemic tissues of CatK−/−mice that received c-Kit+BM MNCs cells of GFP+CatK+/+mice. Scale bar, 50 μm. Figure 8: Blood flow and capillary formation were improved in CatK −/− mice that received CatK +/+ BM-derived EPC-like c-Kit + cells. ( a – c ) In both genotypes of mice, BM-derived c-Kit + EPC-like c-Kit + cells isolated with microbeads (2 × 10 6 per mouse) were injected directly into the BM cavities of both tibias of irradiated CatK −/− mice (9 Gy) (see Supplementary Fig. 15 ) for 40 days. The mice were subjected to ischaemic surgery, after which their blood flow was measured by an laser Doppler blood flow (LDBF) analyser and capillary density was measured by immunofluorescence with fluorescein isothiocyanate-labelled CD31 + antibody. Representative images ( a ) and quantitative data for blood flow recovery (expressed as ischaemia-to-nonischemia LDBF ratio ( b ); and capillary density (expressed as capillary-to-myofibre ratio ( c ). Data are means±s.e.m. ( n =8). * P <0.05 by Student’s unpaired t -test. ( d , e ) CD31 + c-Kit + measured by FACS analysis in BM and PB of CatK −/− mice that received BM transplantation of both genotypes of mice. Representative images ( d ) and quantitative data ( e ) for CD31 + c-Kit + EPC-like cell plots and their percentage in BM and/or PB of both genotypes of mice (counted total 5 × 10 4 cells). Data are means±s.e.m. ( n =6). † P <0.05 by analysis of variance and Tukey’s post hoc tests. ( f ) At day 14 after ischaemic surgery, fluorescence staining with an anti-c-Kit monoclonal antibody (red) showed EPC homing in to the vasculature of the ischaemic tissues of CatK −/− mice that received c-Kit + BM MNCs cells of GFP + CatK +/+ mice. Scale bar, 50 μm. Full size image This study focused on a novel mechanism and molecular requirements for the CatK-mediated close association between Notch1 processing-related signalling transduction and EC/EPC angiogenic actions in ischaemia-induced neovascularization. Our main findings were as follows. (1) In cultured ECs, hypoxia enhanced VEGF-induced CatK expression and activity; and CatK inhibition by genetic or pharmacological interventions impaired proangiogenic activities of mature ECs and EPCs, accompanied by reduced production of c-Notch1 associated with the reduction of Hes1, Hey1, Hey2 and VEGF protein expression as well as of Akt phosphorylation. (2) In vivo , CatK deficiency resulted in decreased BM EPC mobilization and homing in to support ischaemic vasculogenesis associated with the reduction in Notch1-Hes1/Hey1/2 signalling transduction; and impaired vascular action was rescued by cell therapy with CatK +/+ BM-derived c-Kit + EPC-like cells in CatK −/− mice. The mechanisms underlying the impairment of ischaemia-induced neovascularization in CatK −/− mice are schematically represented in Supplementary Fig. 14 . It is well established that the Notch1 receptor is processed in the endoplasmic reticulum/Golgi by furin-like convertase at site S1 during trafficking to the cell surface, producing a heterodimeric surface receptor. Notch1 binding to ligands (DII-1, -4, Jagged-1) expressed on neighbouring cells initiates two successive cleavages by tumour necrosis-α−converting enzyme at site S2 (cell surface), followed by intramembranous cleavage at site S3 by the complex of γ-secretase (reviewed in ref. 19 ). Meanwhile, NICD1 moves into the nucleus to form a transcription complex consisting of the DNA-binding protein and then regulates its downstream targeted gene transcriptions. Here, in vivo , CatK deficiency reduced the levels of c-Notch1 of ischaemic muscles as compared with control. Gene ablation and pharmacological inhibition of CatK impaired Notch1 cleavage in vivo and in vitro . Moreover, CatK overexpression by plasmid promotes c-Notch1 processing and downstream molecule expression in cultured HUVECs. Thus, CatK plays a partial role in the proteolytic processing of NICD1 ( Supplementary Fig. 8 ). This notion was further supported by the sensitivity of the γ-secretase substrate to rhCatK. Given the overlapping substrate specificity of lysosomal proteases, it is notable that CatK seems to be particularly important for EC and EPC transmigration. Previous studies using CatK knockout animals provide evidence that CatK specifically mediates biological effects in cellular events [21] , [30] . In line with these findings, our results showed that blood flow recovery and capillary formation following hindlimb ischaemia were substantially impaired in CatK −/− mice. Moreover, pharmacological inhibition and siRNA interference of CathK impaired EC migration/invasion, proliferation and tubule formation. Among Cat family members, CatS and CatL were shown to contribute to angiogenesis [4] , [12] . However, the pharmacological inhibition of these Cats did not affect the migration or proliferation of mature ECs or vascular smooth muscle cells [12] , [15] . In vitro studies demonstrated that neither elastase inhibition nor MMP inhibition affects mature EC migration and proliferation [2] , [3] . In 2007, we reported that genetic ablation of MMP-2 had no effect on EC or EPC migration [2] . Moreover, Urbich et al . [12] demonstrated that MMP-9-deficient progenitor cells showed no impairment in their ability to augment neovascularization in vivo . In contrast, our observations here show a failure of CatK −/− EPCs to incorporate into the existing endothelial network. Thus, our data indicate that CatK has a specific and crucial role, as opposed to other Cats or MMP-2/MMP-9, in the angiogenic actions of mature ECs and EPC-like mononuclear cells (MNCs) in the neovascularization process. Recently, it was reported that ischaemia-induced Notch1 activation via the VEGF/Akt signalling pathway [17] . In vitro , Notch1 mutation impairs vascular cell and EPC function [17] , [31] . We have shown that genetic ablation and pharmacological inhibition of CatK caused reductions in not only VEGF/VEGFR-1 and p-Akt but also /c-Notch1, Hes1, and Hey1/2 in various vascular cells and ischaemic tissues in response to hypoxia. As compared with the silencing of CatK, plasmid-mediated CatK overexpression enhanced c-Notch1 production. Likewise, hypoxia enhanced VEGF-induced cell-based or ischaemic muscle-based extract-mediated γ-secretase substrate degradation ability; and these effects were abolished by a specific CatK inhibitor. Except for rhCatK, rhMMPs (rhMMP-1, rhMT-MMP-1) and Cats (rhCatS, rhCatB, rhCatV), no MMP or Cat family members can degrade the γ-secretase substrate probe. Moreover, siCatL and CatS plasmid had no effects on Notch1 processing in HUVECs. Collectively, CatK-mediated Notch1 processing and downstream transduction signalling activation appears to represent a novel mechanism in the protection of cardiovascular tissues to hypoxic stress in vivo and in vitro . The impairment of neovascularization in CatK −/− mice may be related to a reduced capacity of EPC to promote vasculogenesis. The data from flow cytometry demonstrated that there were significantly fewer EPC-like CD31 + c-Kit + cells in the PB of CatK −/− mice after ischaemia than in that of CatK +/+ mice. Immunohistochemistry using GFP-green mice confirmed BM-derived EPC-like c-Kit + cells homing in to ischaemic tissues. Moreover, ELISA showed that CatK deficiency significantly reduced plasma VEGF levels at day 7 after ischaemia in CatK −/− mice compared with CatK +/+ mice. VEGF has been shown to modulate EPC mobilization from BM to the circulation and to support vasculogenesis [32] , [33] . More importantly, our observations here show that the reception of CatK +/+ BM-derived EPC-like MNCs, but not that of CatK −/− BM-derived EPC-like MNCs, rescued blood flow impairment after hindlimb ischaemia in CatK −/− mice. Thus far, CatL is the only Cat that has been reported to contribute to ischaemic vasculogenesis [12] . However, genetic or pharmacological inhibition of CatL had no effect on EPC migration and/or mobilization [12] . Moreover, genetic ablation of CatD, a related member of the Cat family, had no effect on the ability of BM-derived stem cells to promote neovascularization following ischaemia [12] . On the basis of these data, in conjunction with the fact that CatK deletion mitigated c-Notch1 processing in EPCs whereas other Cats did not, we can infer that the impairment of vasculogenesis in CatK −/− mice may be attributable to the decrease in EPC mobilization and to its dysfunctional incorporation into the vasculature associated with the impairment of Notch1 cleavage and downstream transduction signalling pathway activation. But the finding that most of our experiments show only partial inhibition of neovascularization by pharmacological or genetic depletion of CatK indicates that other proteases support the incorporation of EPC into the ischaemic limbs. VEGF is essential for developmental and pathological angiogenesis. In 2007, lee and colleagues demonstrated that genetic deletion of VEGF specifically in the endothelial lineage leads progressive endothelial degeneration and sudden death in 55% of mutant mice by 25 weeks mice of age [34] . Recently, we have reported that silencing of VEGF or VEGFR2 enhanced EC apoptosis and proliferation [23] . These results suggest a cell-autonomous VEGF signalling pathway that holds significance for vascular homoeostasis but is dispensable for the angiogenic action. It should be noted that Lee et al . [34] show that in the absence of any pathological insult, autocrine VEGF is required for the vascular homoeostasis. Here, Di et al . [23] reported that VEGFR2 silencing impaired old HUVEC tubulogenesis under hypoxia. Further study will be needed to investigate the role of the autocrine signalling in the angiogenic cascade under pathological ischaemic stress. Several limitations of the present work should be pointed out. First, this study could not fully explore CatK-related bona fide cleavage site in Notch1 and the difference in c-Notch1 processing between γ-secretase and CatK even though several approaches (including genetic silencing, overexpression, pharmacological inhibition of CatK, and so on) have been used to provide direct evidence for CatK-mediated c-Notch1 processing and downstream transduction signalling pathway activation. Second, we also could not show evidence whether CatK is, like tumour necrosis-α converting enzyme, involved in Notch1 processing on the EC surface. In 2006, we demonstrated that, among Cat family members, only active CatS colocalized with integrin ανβ3 as a receptor on the smooth muscle cell surface, playing a key role in cell invasive behaviour [15] . Our observations from the immunofluorescence assay here show that CatK localized in the intramembranous regions and accumulated by VEGF stimulation under hypoxia in cultured HUVECs. These findings suggest that Notch1 processing by CatK is at the intramembranous region rather than the pericellular region. Further study is needed to investigate these issues. Taken together, the previous and present findings show a critical role for CatK in angiogenesis and vasculogenesis. This novel biological function of CatK may be exploited for the therapeutic control of pathophysiological neovascularization. Reagents GM6001 (also known as MMP inhibitor), CatK inhibitor II [1-(N-Benzyloxycarbonyl-leucyl)-5-(N-Boc-phenylalanyl-leucyl)carbohydrazide], CatL inhibitor V [Z-Phe-Tyr(O t Bu)-COCHO · H 2 O], CA-074 (also known as cathepsin B inhibitor III; [L-3- trans - (propylcarbamoyl)oxirane-2-carbonyl]-L-isoleucyl-L-proline), CA-074Me (also known as cathepsin B inhibitor IV; [L-3- trans -(propylcarbamoyl)oxirane-2-carbonyl]-L-isoleucyl-L-proline methyl ester), E64d [(L-3- trans -ethoxycarbonyloxirane-2-carbonyl)-L-leucine (3-methylbutyl) amide], and E64 (N-[N-(L-3-Trans-carboxirane-2-carbonyl)-L-leucyl]-agmatine) were purchased from Calbiochem (San Diego, CA, USA). DAPT [also known as γ-secretase inhibitor IX; (3,5- difluorophenylacetyl)-L-alanyl-L-2-phenylglycine t -butyl ester], L-685,458 (also known as γ-secretase inhibitor X; [(2 R ,4 R ,5 S )-2-benzyl-5-( t -butyloxycarbonylamino)-4-hydroxy-6-phenylhexanoyl]-L-leucyl-L-phenylalanine amide), and fluorescence-quenching substrate (also known for γ-secretase; Nme-Asp-Gly-Cys-Gly-Val-Leu-Leu-Lys-DNP-Arg-Arg-NH2) were purchased from the Peptide Institute (Osaka, Japan). All powdered reagents were dissolved in sterilized dimethyl sulfoxide (DMSO) and added to the cell culture medium to yield 0.2% DMSO as a final concentration. Animals and model of hindlimb ischaemia The Nagoya University Graduate School of Medicine Animal Care and Use Committee approved this study. Male CatK knockout mice (KO, CatK −/− ) [35] and wild-type (CatK +/+ ) littermates (8 weeks of age) were subjected to unilateral hindlimb ischaemic surgery under sodium pentobarbital anaesthesia (50 mg kg − intraperitoneally). In the specific experiments, a specific CatK inhibitor, CatK-II (5 mg kg −1 ; Sigma-Aldrich, St Louis, MO, USA), dissolved in dimethyl sulfoxide (CatK-II group) or vehicle (control group) alone, was injected into the abdomen of CatK +/+ mice ( n =6 in each group) every other day from 3 days prior to surgery until 14 days after surgery. The animals were euthanized by an overdose of sodium pentobarbital at indicated time points after surgery. Skeletal muscles were dissected out and immediately frozen in liquid nitrogen. Ischaemic hindlimb perfusion assay At the indicated time points, the ratio of ischaemic blood flow (left) to that in the normal (right) limb was measured with a laser Doppler blood flow imager (Lisca AB, Jarfalla, Sweden). After blood flow was scanned twice, stored images were subjected to computer-assisted quantification, and the average flows of ischaemic and nonischemic limbs were calculated. Capillary density At day 28, capillary ECs in each cross-cryosection (6 μm) were evaluated with anti- Griffonia simplicifolia -lectin-1 (GSL-1, Vector Laboratories) [2] . The capillaries and muscle fibres were counted in five random microscopic fields from three independent cross-sections of the adductor skeletal muscle in each animal ( n =6 per group), and then capillary density was expressed as the number of capillaries per muscle fibre (× 200). Western blot analysis Protein was extracted using a RIPA lysis buffer and western blotted against antibodies for VEGF, total Notch1 (t-Notch1), c-Notch1 and presenilin 1 (carboxy-terminal antibody); total Akt (t-Akt), p-Akt, Hes1, Ephrin B2 and Flk-1 (Cell Signaling Technology, Boston, MA, USA); Jagged-1 and Flt-1 (Santa Cruz Biotechnology, Santa Cruz, CA, USA); human laminin-5 (Bioss, Woburn, MA, USA), Hey1 and Hey2 (Proteintech, Chicago, IL, USA) and β-actin (Sigma-Aldrich; loading control) (1:1000 for each antibody) [18] . Full scans of immunoblots, PCR and zymography gels are shown in Supplementary Fig. 16 . Quantitative real-time gene expression assay RNA was harvested from tissue with an RNeasy Fibrous Tissue Mini Kit and from cultured cells with an RNeasy Micro Kit (Qiagen, Hilden, Germany) in accordance with the manufacturer’s instructions. The mRNA was reverse-transcribed to cDNA with an RNA PCR Core kit (Applied Biosystems, Foster City, CA, USA). Quantitative gene expression was studied using the ABI 7300 real-time PCR system with Universal PCR Master Mix (Applied Biosystems). All experiments were performed in triplicate. The sequences of primers for the targeted genes were described in Supplementary Table 2 (refs 2 , 36 ). The transcription of targeted genes was normalized to glyceraldehyde 3-phosphate dehydrogenase. Full scans of immunoblots, PCR and zymography gels are shown in Supplementary Fig. 16 . Levels of VEGF protein At 7 days after surgery, the contents of human VEGF165, basic fibroblast growth factor, endostatin, tumour necrosis factor-α and interleukin-1β in mouse plasma and ischaemic tissues ( n =6 for each time point) were measured using a commercially available ELISA kit (R&D Systems, Minneapolis, MN, USA) according to the manufacturer’s instructions. Acidic gelatin zymography Equal amounts of total protein (40 μg) were mixed with SDS sample buffer without a reducing agent and loaded onto a 12.5% SDS polyacrylamide gel containing 0.2% gelatin at 4 °C (ref. 20 ). Gels were then incubated in activity buffer (0.1 M sodium phosphate buffer, pH 6.0, 1 mM EDTA and 2 mM DTT freshly added) overnight at 37 °C. For different pH conditions, 0.1 M sodium acetate buffers of pH 4 and sodium phosphate buffers of pH 6, 7 and 8 were used. Following Coomassie staining, digestion bands were quantified by an image analyser system (NIH Image 1.62). Data were representative of at least five independent experiments. Full scans of immunoblots, PCR and zymography gels are shown in Supplementary Fig. 16 . Assay for γ-secretase activity The assay for γ-secretase activity was performed as described previously [37] . Briefly, the extracts of the muscles were incubated with 8 μmol l −1 of intramolecularly quenched fluorogenic peptide probe, harbouring the substrate for γ-secretase (Enzo Life Sciences, Farmingdale, NY, USA) in buffer containing 50 mM sodium acetate, pH 6.8, 2.5 mM EDTA, 0.01% Triton X-100 and 1 mM DTT for 24 h. Twenty micromoles per liter of fluorogenic peptide probe was also incubated with recombinant human CatS, CatB, CatL, CatV and CatK (R&D Systems) or with matrix metalloproteinase-1 (MMP-1), membrane-type 1 of MMP (Enzo Life Sciences) in the presence or absence of the related protease inhibitors at their respective optimal pH conditions. Fluorescence was measured using a plate reader (Fluoroskan Ascent CF, Labsystems) with an excitation wavelength of 355 and an emission wavelength of 440 nm (ref. 17 ). Endothelial explant assay This ex vivo angiogenesis assay was performed essentially as described previously [2] . The rings from the descending thoracic aortas of CatK −/− and CatK +/+ mice were inserted between two layers of type I collagen gel (BD Biosciences, Franklin Lakes, NJ, USA) and cultured in endothelial cell basal medium-2 (EBM-2) (Chambrex, East Rutherford, NJ, USA) containing 50 ng ml −1 VEGF (Genzyme/Techne) in the presence or absence of specific protease inhibitors for 10 days [2] . Microvascular sprouting was characterized by the incorporation of 1,1′-dioctadecyl-3,3,3′3′-tetramethylidocarbocyanine perchlorate-labelled acetylated low density lipoprotein (Dil-acLDL, 10 μg ml −1 , Molecular Probes, Eugene, OR, USA). To further confirm that outgrowing structures have capillaries features, as previously studied in human aorta-ring culture assays [22] , we also examined sprouting cells by immunostaining and confocal microscopy using fluorescein isothiocyanate-labelled CD31 monoclonal antibody (BM Pharmingen). Sprout length was quantified using BZ-II Analyser, Exe 1.42 software (Keyence, Osaka, Japan). Endothelial cell sprouting density was expressed as a percentage of pixels per image occupied by vessels within a defined area. Cell culture HUVECs, ECs and RAECs were purchased from Cell Applications (San Diego, CA, USA) and cultured in EBM-2 plus 10% fetal bovine serum and EGM-2 SingleQuotes (Clonetics, San Diego, CA, USA) in a humidified atmosphere of 5% CO 2 and 95% air. Mouse pulmonary ECs were isolated from CatK −/− and CatK +/+ mice by a protocol using PECAM-1-coated Dynabeads (Invitrogen Life Technologies, Carlsbad, CA, USA) and then were cultured in EGM-2 (ref. 38 ). The isolated ECs retain their in vivo characteristics (purity>85%), such as the expression of cell surface marker PECAM-1 and intracellular adhesion molecule-2. After passage by trypsinization, the cells were cultured in serum-free medium overnight and then treated with 20 ng ml −1 VEGF and/or 400 μM CoCl 2 containing the following reagents for the indicated times: CA-074Me (10 μM); E64 d (10 μM); CatK inhibitor II, CatL inhibitor V, GM6001 and CatG inhibitor I (10 μM); DAPT (1 μM); and L-685,458 (1 μM). The ECs were also cultured under normoxic (5% CO 2 and 95% air) and hypoxic (2% O 2 , 5% CO 2 and 93% N 2 ) conditions for testing on the effects of mechanical hypoxia on Notch1 processing. Silencing and overexpression of Cats CatK-specific siRNAs (#F5129442005, #F5129442006), CatL-specific siRNAs (#F55214357-001/2, #F55214357003/4) and nontargeting control siRNA (#F5129292-921) were purchased from Sigma-Aldrich (St Louis, MO, USA). Briefly, cells were grown on 60-mm dishes until 80% confluence. The siRNA solution mixed with serum-free and antibiotic-free EBM-2 medium containing Lipofectamine Transfection reagent (Invitrogen Life Technologies) was added to each well to achieve a final siRNA concentration of 100 pM. The cells were incubated at 37 °C for 48 h, and the levels of targeted gene and protein were analysed by PCR and WB. Transfected cells were also used for cellular functional experiments. Silamin A/C (D0010500105; Dharmacon, Brébières, France) was used as a positive control [39] . For overexpression experiments, CatK plasmid or CatS plasmid (both from Invitrogen) was transformed in competent Escherichia coli cells by using the heat shock method, followed by purification using a Qiagen plasmid mini kit (Qiagen) [40] . CatK and CatS plasmids were then transformed in HUVECs with the help of lipofectamine LTX & Plus reagents according to the manufacturer’s instructions (Invitrogen). Cell migration and invasion assays Migration and invasion assays were performed on Transwell (Costar) 24-well tissue culture plates as previously described [2] . The cells that migrated and invaded to the outer side of the membrane were stained and counted in six to eight randomly chosen fields of the duplicated chambers at a magnification of × 200 for each sample. Cell proliferation assay Endothelial cell proliferation was assessed with the Cell Titer 96AQ Assay kit (Promega, Madison, WI, USA) [23] . Cells were plated on collagen-coated 96-well plates at 5,000 cells in 100 μl of 0.3% bovine serum albumin/DMEM per well and incubated with EBM-2 in the presence of VEGF (50 ng ml −1 ) for 24 h. Then, 20 μl of a mixture of tetrazolium compound and phenazine methosulfate was added, and the absorbance was determined at 492 nm. Experiments were performed five separate times for each group in triplicate. Immunocytofluorescence After the attachment of HUVECs (cell density at 2 × 10 4 cells per well) to coverslips precoated with gelatin, the cells were cultured under normoxic (5% CO 2 and 95% air) and hypoxic (2% O 2 , 5% CO 2 and 93% N 2 ) conditions in the presence or absence of VEGF (50 ng ml −1 ) overnight. Then, the cells were fixed for 10 min with 8% paraformaldehyde and washed with 1% glycerol. Following blocking with 0.1% bovine serum albumin/phosphate-buffered saline, the cells were studied by immunofluorescence as described previously [23] . Coverslips were treated with Prolong mounting medium (Molecular Probes) and visualized by confocal microscopy. Analysis of EPCs At day 10 after ischaemic surgery, following treatment with mouse anti-CD16 + and CD32 + mAb, EPC-like MNCs in both PB and BM were identified by flow cytometry using antibodies to CD31 + or CD34 + and c-Kit + (BM Pharmingen) [2] . BM transplantation BM transplantation was performed in two groups of young mice (8 weeks old; n =5 per group): CatK +/+ donor/CatK −/− recipient and CatK −/− donor/CatK −/− recipient. Following BM harvesting from femurs and tibias, BM-derived EPC-like c-Kit + MNCs isolated with microbeads (2 × 10 6 per mouse) were injected directly into the BM cavities of both tibia of irradiated mice (9 Gy) ( Supplementary Fig. 15 ) [41] . After allowing 40 days for BM reconstitution, the mice were subjected to ischaemic surgery. Statistical analysis Data are expressed as means±s.e. Student’s t -test (for comparison between groups) or one-way analysis of variance (for comparison of three or more groups) followed by Tukey’s post hoc tests were used for statistical analyses. Blood flow data were subjected to two-way repeated measures analysis of variance and Bonferroni’s post hoc tests. Collateral capillary density, length and number of endothelial sprouts were evaluated by two observers in a blind manner, and the values they obtained were averaged. SPSS software version 17.0 (SPSS, Chicago, IL, USA) was used. A value of P <0.05 was considered statistically significant. How to cite this article: Jiang, H. et al . Cathepsin K-Mediated Notch1 activation contributes to neovascularization in response to hypoxia. Nat. Commun. 5:3838 doi: 10.1038/ncomms4838 (2014).